Clonal culturing of human embryonic stem cells on laminin-521/E-cadherin matrix in defined and xeno-free environment Lack of robust methods for establishment and expansion of pluripotent human embryonic stem (hES) cells still hampers development of cell therapy. Laminins (LN) are a family of highly cell-type specific basement membrane proteins important for cell adhesion, differentiation, migration and phenotype stability. Here we produce and isolate a human recombinant LN-521 isoform and develop a cell culture matrix containing LN-521 and E-cadherin, which both localize to stem cell niches in vivo . This matrix allows clonal derivation, clonal survival and long-term self-renewal of hES cells under completely chemically defined and xeno-free conditions without ROCK inhibitors. Neither LN-521 nor E-cadherin alone enable clonal survival of hES cells. The LN-521/E-cadherin matrix allows hES cell line derivation from blastocyst inner cell mass and single blastomere cells without a need to destroy the embryo. This method can facilitate the generation of hES cell lines for development of different cell types for regenerative medicine purposes. Human stem cells hold promise for the development of regenerative medicine for a variety of degenerative diseases and injuries. Optimally, development of stem cell–derived cell therapies requires methods that enable derivation and long-term genetically stable pluripotent stem cells growth under chemically defined and xeno-free conditions. Generally, human embryonic stem (hES) and induced pluripotent stem (iPS) cells have been cultured on various feeder cell layers [1] , [2] or Matrigel [3] that are chemically undefined batch-to-batch variable substrata, but recently, several groups have reported new cell culture matrices that allow robust self-renewal of hES and iPS cells. Thus, we [4] and other investigators [5] , [6] have developed completely chemically defined xeno-free cell culture systems for self-renewal of human pluripotent cells. We have shown that human recombinant LN-511, expressed in the blastocyst inner cell mass, alone can support monolayer cultures and self-renewal of both mouse ES [7] and human pluripotent ES and iPS cells [4] . Laminins are a large family of heterotrimeric basement membrane adhesion proteins that are highly cell and tissue type specific [8] . These heterotrimers consist each of one α, one β and one γ chain, the proteins being named according to the chain composition (for example LN-521 consists of α5, β2 and γ1 chains) [9] . To date, at least 16 laminin isoforms are known to exist in mammalian tissues, and most of them have been produced in our laboratory as recombinant proteins [10] , [11] . Other investigators have reported that recombinant vitronectin [12] , a hydrogel [13] , and a LN-511 fragment [14] can serve as alternatives to Matrigel or feeder cells for culturing of hES cells. However, none of the cell culture substrata allows clonal survival of hES cells without the use of apoptosis inhibitors [15] , [16] , [17] or chemically undefined substances [18] , [19] , and the cells are often passaged in small clumps that can contain a significant proportion of differentiated cells. Since the initial number of cells is low during derivation of new ES cell lines, absence of cell culture conditions that enable clonal survival also complicates the derivation procedure especially from single blastomeres. Indeed, there is still a lack of robust methods for derivation of new hES cell lines under chemically defined and xeno-free conditions despite significant advances in culturing of pluripotent hES cells. Also a method for clonal derivation of hES cells under fully defined xeno-free conditions has not been reported. Originally, hES cells were established and cultured on a layer of mitotically inactivated mouse fibroblasts in media containing fetal calf serum [1] . Despite drawbacks concerning system complexity, feeder cell layers are still widely used [20] , [21] , [22] , [23] , although they can be sources of viral and bacterial contaminations. Moreover, undefined and day-to-day batch-to-batch variable amounts of proteins and small molecules produced by the feeder cells can interfere with scientific studies and developed clinical procedures in unpredictable ways. Only one group has reported derivation of two lines under xeno-free feeder-free, but not chemically defined conditions, and both those lines eventually became genetically abnormal [24] . In the present study, we sought to identify natural conditions that allow clonal survival and self-renewal of hES cells. We produced as human recombinant proteins all the laminin isoforms known to be expressed in hES cells and tested them for ability to support hESC cell self-renewal in vitro . Apart from previously described LN-511, only LN-521 can support long-term self-renewal of the cells in completely defined and xeno-free environment but, unlike LN-511, permits survival of individualized human ES/iPS cell plated at certain densities. Time-lapse imaging of hES cells plated from single-cell suspensions reveals that LN-521 alone does not support their clonal derivation and self-renewal, and that the cells appear to require migration and cell–cell contact for the proliferation. We, therefore, explored if E-cadherin, a cell–cell receptor expressed by cells of the ICM, could support clonal expansion, and discovered that only LN-521 and E-cadherin together as a culture matrix support both derivation and clonal survival of hES cells. We also demonstrate that a single cell obtained by biopsy from an 8-cell human in vitro fertilized (IVF) embryo can give rise to new hES cell lines under completely chemically defined and xeno-free conditions. The methods developed here may have significance for research and clinical applications of hES cells. Effects of human laminin isoforms on human stem cells We and others have already shown that pluripotent hES cells express α1, α5, β1, β2 and γ1 laminin chains [4] , [25] , suggesting that the cells express four laminin isoforms LN-511, LN-521, LN-111 and LN-121. Of those, α5 chain laminins are found in stem cell niches of blastocysts (inner cell mass) [26] , hair follicles [27] and intestinal villus crypts [28] . To study the properties of those isoforms as in vitro culture substrata for ES/iPS cells, we cloned the laminin chains and produced these laminins as recombinant human proteins, essentially as described in refs 10 , 11 ( Supplementary Fig. 1 ). To compare the survival of hES cells on different culture substrata, we plated dissociated cells in single-cell suspension on Matrigel, LN-111, LN-121, LN-511 and LN-521 or on a mixture of the latter two, in the absence or presence of a ROCK inhibitor (Y-27632) at a density of 40,000 cells per 1 cm 2 , and analysed the cultures after 24 h. As shown in Fig. 1a , the cells did not survive well on Matrigel or LN-111, but they did readily adhere and spread on human recombinant LN-511 and LN-521, as well as on a mixture of the two. They did not survive on LN-121. With ROCK inhibitor, the hES cells survived on all surfaces, but there were clear differences with regard to cell shapes between cells growing in the absence or presence of ROCK inhibitor ( Fig. 1b ). 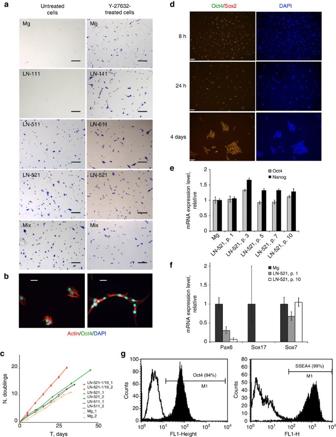Figure 1: Survival and long-term self-renewal of dissociated hES cells on human recombinant laminins and Matrigel. (a) Crystal Violet staining of hES cells 24 h after plating cells (40,000 cells per cm−2) in single-cell suspensions onto Matrigel (Mg), LN-111, LN-511, LN-521, and an equal mixture of LN-511/LN-521 (mix) without (untreated cells) and with 10 μM of Y-27632 (treated cells). Magnification × 5. Scale bar, 250 μm. (b) Immunostaining of hES cells 24 h after plating from single-cell suspensions onto LN-521 without (left panel) and onto Matrigel with Y-27632 (right panel). Oct4 (green); DAPI (blue); rhodamine phalloidin (Actin, red). Scale bars, 27 μm. (c) Growth curves of HS181 hES cells cultured on LN-521 passaged as single cells in 1:10 ratio (red) and in 1:20–1:30 ratios (green); and on LN-511 (black); and on Matrigel passaged in pieces (orange). After the experiment, the cells were immunostained to confirm Oct4 expression. Two independent experiments were performed per each condition. (d) Immunostaining of HS181 hES cells for pluripotency markers Oct4 and Sox-2 8 h, 24 h and 4 days after plating of dissociated cells onto LN-521. Right panels show DAPI staining. Scale bars, 110 μm. (e) Quantitative reverse transcriptase polymerase chain reaction analysis shows relative amounts of mRNA transcripts for pluripotency markers at different time points (1, 3, 5, 7 and 10 passages) in HS181 hES cells cultured on LN-521 and in the control cells on Matrigel. All reactions were done in quadruplicates. Error bars show 95% confidence intervals. (f) Same for differentiation markers Pax6, Sox17 and Sox7. All reactions were done in quadruplicates. Error bars show 95% confidence intervals. (g) FACS analysis of hES cells after 15 passages on LN-521 for markers of pluripotency. The percentage of positive cells is listed in parentheses. In the absence of ROCK inhibitor, the cells failed to survive on any coating after plating at densities lower than 5,000 cells per cm 2 Figure 1: Survival and long-term self-renewal of dissociated hES cells on human recombinant laminins and Matrigel. ( a ) Crystal Violet staining of hES cells 24 h after plating cells (40,000 cells per cm −2 ) in single-cell suspensions onto Matrigel (Mg), LN-111, LN-511, LN-521, and an equal mixture of LN-511/LN-521 (mix) without (untreated cells) and with 10 μM of Y-27632 (treated cells). Magnification × 5. Scale bar, 250 μm. ( b ) Immunostaining of hES cells 24 h after plating from single-cell suspensions onto LN-521 without (left panel) and onto Matrigel with Y-27632 (right panel). Oct4 (green); DAPI (blue); rhodamine phalloidin (Actin, red). Scale bars, 27 μm. ( c ) Growth curves of HS181 hES cells cultured on LN-521 passaged as single cells in 1:10 ratio (red) and in 1:20–1:30 ratios (green); and on LN-511 (black); and on Matrigel passaged in pieces (orange). After the experiment, the cells were immunostained to confirm Oct4 expression. Two independent experiments were performed per each condition. ( d ) Immunostaining of HS181 hES cells for pluripotency markers Oct4 and Sox-2 8 h, 24 h and 4 days after plating of dissociated cells onto LN-521. Right panels show DAPI staining. Scale bars, 110 μm. ( e ) Quantitative reverse transcriptase polymerase chain reaction analysis shows relative amounts of mRNA transcripts for pluripotency markers at different time points (1, 3, 5, 7 and 10 passages) in HS181 hES cells cultured on LN-521 and in the control cells on Matrigel. All reactions were done in quadruplicates. Error bars show 95% confidence intervals. ( f ) Same for differentiation markers Pax6, Sox17 and Sox7. All reactions were done in quadruplicates. Error bars show 95% confidence intervals. ( g ) FACS analysis of hES cells after 15 passages on LN-521 for markers of pluripotency. The percentage of positive cells is listed in parentheses. Full size image Self-renewal of hES cells on laminin-521 To test if LN-521 could be used alone as a cell coating material for long-term self-renewal of human pluripotent stem cells, we cultured three hES cell lines, HS181, HS401, H1 and human iPS ChiPSW and CVTB1.2 cells on this protein in O3, mTeSR1 or TeSR2 media. The cells could be passaged in single-cell suspensions at ratios of 1:20–1:30 to acquire large numbers of pluripotent cells at a time or at ratio of 1:10 to provide the fastest multiplication of the cell number ( Fig. 1c ). In the latter case, the cells were passaged every 5–6 days. By now, HS181, HS401 and H1 cells have proliferated for 37, 25 and 35 passages, respectively (12, 8 and 11 months), in O3 or mTeSR1 medium ( Supplementary Table 1 ). CVTB1.2 iPS and ChiPSW iPS cells have been cultured for 15 and 10 passages in mTeSR1, respectively. Importantly, dissociated hES cells could be cultured and passaged on LN-521 under chemically defined and xeno-free conditions, using TeSR2 medium and TrypLE Select enzyme. By now, the H1 and HS401 cells have been cultured for 14 and 12 passages, respectively (5 and 4 months), in TeSR2. On LN-521, the cells grew in monolayers and showed stable expression levels of the pluripotency markers Oct4, Nanog, Sox2 ( Fig. 1d,e,g and Supplementary Fig. 2a,b ), and SSEA4 ( Fig. 1g and Supplementary Fig. 2c ), which were similar to those in cells plated on Matrigel and passaged in small clumps. Additionally, quantitative reverse transcriptase polymerase chain reaction revealed similar or lower levels of expression of the differentiation markers PAX6, SOX17 and SOX7 in LN-521 cultures as those in the control cells grown on Matrigel ( Fig. 1f ). Karyotypes were confirmed to be normal for hES cell lines HS181 and H1 after 29 and 31 passages, respectively, ( Supplementary Fig. 3 ), and for H1 after seven passages in TeSR2 medium. Histological examination of teratomas formed in severe combined immunodeficiency (SCID) mice after injection of HS181 and H1 cells cultured for 29 and 12 passages, respectively, on LN-521 in O3 medium, and H1 cells cultured for 7 passages on LN-521 in TeSR2 revealed development of tissues containing cell lineages of all three embryonic germ layers ( Supplementary Fig. 4a–f ). Differentiation in vitro also revealed that cells of all the three hES cell lines retained the competence to form embryoid bodies expressing markers of mesoderm (smooth-muscle actin), ectoderm (MAP-2) and endoderm (α-fetoprotein) ( Supplementary Fig. 4g ). LN-521 interaction with α6β1 integrin in hES cell self-renewal To quantify the effect of laminins, we studied adhesion after 1 h and survival after 24 h of dissociated hES cells on Matrigel, LN-111, LN-511, LN-521 and an equal mixture of the latter two. Interestingly, after 1 h, the same 75–80% of cells had adhered to all the coatings ( Fig. 2a ), but spreading of the cells was clearly better on LN-521 and LN-511 than on Matrigel or LN-111. After 24 h, almost no cells had survived on Matrigel, LN-111 or LN-121, but some on LN-511. In contrast, hES cells thrived well on LN-521 ( Fig. 2b ). To qualitatively compare the effects of LN-521 and the ROCK inhibitor, we plated cells from a single-cell suspension at the same plating density in a medium with or without Y-27632 on the different coatings ( Fig. 2b ). The untreated cells on LN-521 and Y-27632-treated cells on Matrigel showed similar survival rate 24 h after plating. If exogenous bFGF was not included in the O3 medium, the cells still survived on LN-521, but not on Matrigel ( Fig. 2c ). 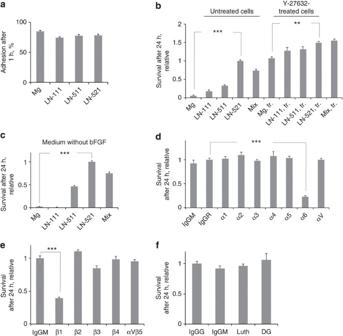Figure 2: Survival of dissociated hES cells on different substrata and role of cell surface receptors. Error bars show s.e.m. (n=4). Statistical significance (P) was calculated by the Student’st-test: ***P<0.002; **P<0.02. (a) Adhesion of hES cells to Matrigel and laminins 1 h after plating. Values are shown as average percentages of cells that stayed attached. (b) Survival of dissociated hES cells on the same coatings and on an equal mixture of LN-511/LN-521 (mix) in O3 medium (untreated cells) and in O3 medium with 10 μM of Y-27632 24 h after plating. Values shown are normalized to survival on LN-521 in O3 medium without additives. (c) Survival of dissociated hES cells on the same coatings in O3 medium without bFGF or Y-27632 24 h after plating. (d–f) Inhibition of survival by integrin and non-integrin function blocking antibodies of hES cells plated on LN-521 (24 h after plating). Bars represent survival of control HS181 cells treated with mouse, rabbit or goat IgG (IgGM, IgGR and IgGG, respectively) taken as standard values to compare and survival of the cells treated with antibodies to human integrin α subunits (α1–α6 and αV), β subunits (β1–β4), Lutheran receptor (Luth) and α-dystroglycan (DG). Figure 2: Survival of dissociated hES cells on different substrata and role of cell surface receptors. Error bars show s.e.m. ( n =4). Statistical significance ( P ) was calculated by the Student’s t -test: *** P <0.002; ** P <0.02. ( a ) Adhesion of hES cells to Matrigel and laminins 1 h after plating. Values are shown as average percentages of cells that stayed attached. ( b ) Survival of dissociated hES cells on the same coatings and on an equal mixture of LN-511/LN-521 (mix) in O3 medium (untreated cells) and in O3 medium with 10 μM of Y-27632 24 h after plating. Values shown are normalized to survival on LN-521 in O3 medium without additives. ( c ) Survival of dissociated hES cells on the same coatings in O3 medium without bFGF or Y-27632 24 h after plating. ( d – f ) Inhibition of survival by integrin and non-integrin function blocking antibodies of hES cells plated on LN-521 (24 h after plating). Bars represent survival of control HS181 cells treated with mouse, rabbit or goat IgG (IgGM, IgGR and IgGG, respectively) taken as standard values to compare and survival of the cells treated with antibodies to human integrin α subunits (α1–α6 and αV), β subunits (β1–β4), Lutheran receptor (Luth) and α-dystroglycan (DG). Full size image An assay for the inhibition of cell survival using function-blocking antibodies to potential laminin receptors on the plasma membrane showed that antibodies to integrins α6, and to a slightly lesser extent to β1, inhibited the survival of human ES cells on LN-521 ( Fig. 2d,e ). Function-blocking antibodies against other integrin subunits, against Lutheran receptor or against α-dystroglycan, showed very little, if any, effects on the survival ( Fig. 2f ). High β1 integrin-dependent motility of hES cells on LN-521 Recently, it has been shown that ROCK inhibitors act through abrogation of actin-myosin contractility [16] , which is mediated by phosphorylation of the myosin light chain (MLC). To test if LN-521 has similar activity, we compared the levels of phosphorylated MLC in dissociated cells growing on Matrigel, LN-111, LN-511 and LN-521 1 and 6 h after plating ( Fig. 3a,b and Supplementary Fig. 5 ). Interestingly, western blotting showed that the phosphorylation of MLC in cells grown on LN-511 and LN-521 was the same as or higher than in cells growing on Matrigel and LN-111. Since actin–myosin rearrangements are also essential for cell motility [29] , we surmised that the cells might survive on LN-521 through fast migration to each other. Time-lapse imaging of the cells on Matrigel ( Supplementary Movie 1 ) and LN-521 ( Supplementary Movie 2 ) revealed that the cells migrate much faster on the latter, rapidly forming small moving monolayer aggregates. Motility of the hES cells on LN-521 was higher than that of the cells on other substrata and it correlated with the survival of the cells ( Fig. 3c ). Treatment with function blocking antibodies against integrin β significantly reduced motility ( Fig. 3d ) and adhesion of the cells on LN-521 ( Fig. 3e ). 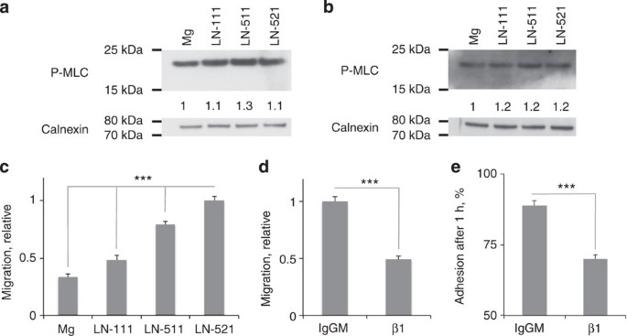Figure 3: Mechanism of dissociated hES cell survival on LN-521. (a) Western blot analysis of phosphorylated MLC (P-MLC) in dissociated HS181 cells 1 h after plating on different substrata. Numbers below P-MLC blot represent quantification of P-MLC signals using Calnexin signals for normalization of the sample input. (b) Same 6 h after plating. (c) Migration of HS181 cells on different coatings. Error bars show s.e.m. (n=100).Pvalue was calculated by Student’st-test: ***P<0.002. (d) Migration of the cells on LN-521 after treatment with integrin function blocking antibodies. Scale bars represent migration of control HS181 hES cells treated with mouse IgG (IgGM) taken as standard values to compare migration of the cells treated with antibodies to human integrin β1 subunit. Error bars show s.e.m (n=100).Pvalue was calculated by Student’st-test: ***P<0.002. (e) Adhesion of hES cells to LN-521 1 h after plating. Values are shown as average percentages of cells that stayed attached. Scale bars represent adhesion of control cells treated with mouse IgG (IgGM) taken as standard values to compare and adhesion of the cells treated with antibodies to human integrin β1 subunit. Error bars show s.e.m (n=100).P-value was calculated by Student’st-test: ***P<0.002. Figure 3: Mechanism of dissociated hES cell survival on LN-521. ( a ) Western blot analysis of phosphorylated MLC (P-MLC) in dissociated HS181 cells 1 h after plating on different substrata. Numbers below P-MLC blot represent quantification of P-MLC signals using Calnexin signals for normalization of the sample input. ( b ) Same 6 h after plating. ( c ) Migration of HS181 cells on different coatings. Error bars show s.e.m. ( n =100). P value was calculated by Student’s t -test: *** P <0.002. ( d ) Migration of the cells on LN-521 after treatment with integrin function blocking antibodies. Scale bars represent migration of control HS181 hES cells treated with mouse IgG (IgGM) taken as standard values to compare migration of the cells treated with antibodies to human integrin β1 subunit. Error bars show s.e.m ( n =100). P value was calculated by Student’s t -test: *** P <0.002. ( e ) Adhesion of hES cells to LN-521 1 h after plating. Values are shown as average percentages of cells that stayed attached. Scale bars represent adhesion of control cells treated with mouse IgG (IgGM) taken as standard values to compare and adhesion of the cells treated with antibodies to human integrin β1 subunit. Error bars show s.e.m ( n =100). P -value was calculated by Student’s t -test: *** P <0.002. Full size image Induction of the PI-3K/Akt pathway in hES cells on LN-521 Extensive body of data has shown that activation of the MEK1/Erk or PI3-kinase/Akt pathways by integrins can block anoikis [30] , [31] , [32] , [33] . Blockade of Akt activation by a specific inhibitor LY 294002 was found to facilitate detachment and hES cell death, with only few cells surviving 24 h after plating on LN-521 ( Supplementary Fig. 6a,b ). In contrast, treatment with PD 98059, a specific inhibitor of MEK1/Erk, did not significantly affect the survival either in the presence or absence of exogenous bFGF. The cells formed similar numbers of monolayer colonies as in the control, but the average size of them was smaller, probably due to the negative influence of the inhibitor on cell proliferation ( Supplementary Fig. 6a–e ). Human ES cells treated with another PI3K/Akt specific inhibitor, Wortmannin, also failed to survive 24 h after plating on LN-521, confirming that the activation of PI3K/Akt was necessary for the cell survival on LN-521 ( Supplementary Fig. 6b ). Western blot analysis of extracts from cells growing on Matrigel and LN-521 with antibodies against phospho-Akt showed that the PI3K/Akt pathway was active in both cases ( Supplementary Fig. 6f ). To determine the levels of Akt activation in the cells on different substrata, we carried out an enzyme-linked immunosorbent assay (ELISA) on cell lysates collected 1 h after plating on Matrigel, LN-111, LN-511 and LN-521 when the cells still did not have direct contacts with each other ( Supplementary Fig. 6g,h ). Clonal survival of hES cells on LN-521/E-cadherin substratum Dispersed, unattached pluripotent cells die from anoikis [16] , which can be prevented by integrin-mediated ECM signalling and cadherin-mediated cell–cell signalling. E-cadherin has been shown to support self-renewal of hES cells if they are passaged in pieces [34] and it is important for reprogramming of somatic cells into iPS cells [35] . Also, it has been reported that laminin and E-cadherin signalling are required for clonal survival of human ES cells [36] and upregulation of E-cadherin expression in human ES cells increases their clonogenicity [37] . To test if E-cadherin was involved in the survival of the cells on LN-521, we employed function-blocking E-cadherin antibodies. Interestingly, while the adhesion to LN-521 was not affected ( Fig. 4a ), we observed that treatment with E-cadherin antibodies significantly decreased the number of cells that had survived 24 h after plating ( Fig. 4b ). We surmised that a mixture of LN-521 and E-cadherin might mimic a natural stem cell niche and permit the clonal survival of human ES cells. To test this, we plated HS181 and H1 cells on LN-521/E-cadherin mixtures with various w/w ratios at cloning densities (150 cells per cm 2 ). Interestingly, neither LN-521 nor E-cadherin alone could provide any significant cloning efficacy of hES cells. The most efficient colony formation was detected on the mixtures of LN-521 and E-cadherin between w/w ratios 10:1 and 5:1. To enhance the effect, we supplemented standard mTeSR1 medium with additional 20 mg ml −1 of bovine albumin. In this medium on LN-521/E-cadherin 9:1 coating mixture, the cloning efficacy of the cells of both lines was around 20% ( Fig. 4c,d ). The use of the ROCK inhibitor on HS181 cells led to a cloning efficacy 14% ( Fig. 4d ). TeSR2 medium supplemented with recombinant human serum albumin supported a similar cloning efficacy, thus allowing survival of individualized hES cells in completely xeno-free and chemically defined environment. Time-lapse photography confirmed that the environment facilitated colony formation through the proliferation of single cells rather than cell aggregates ( Supplementary Movie 3 ). Interestingly, the additional albumin also increased the cloning efficacy on pure LN-521 and to lesser extent on LN-511, but it was still low. Combination of vitronectin with E-cadherin could not support efficient cloning of the cells ( Fig. 4d ). Very few, if any, colonies survived on E-cadherin or Matrigel alone, neither with nor without additional albumin ( Fig. 4d ). To further investigate this, using serial dilutions, we plated approximately one cell of HS181 line per well on 96-well plates under conditions for clonal survival on several substrata ( Table 1 ). Visual microscopic observation was used to identify and count wells containing only one cell. Seven days later, the cells were fixed and stained. The results confirmed high efficacy of hES cell cloning on LN-521/E-cadherin. Three clones of HS181 cells had proliferated and their pluripotency was confirmed in in vitro assays ( Supplementary Fig. 7a ). The cloning experiments were also repeated with hES cells of early passages (HS980 and HS1001, Fig. 4e and Table 1 ) yeilding similar levels of cloning efficacies on LN-521/E-cadherin and other substrata. 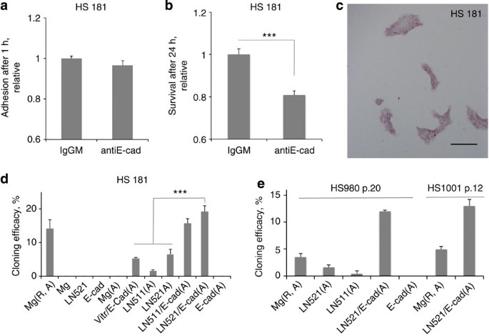Figure 4: Importance of E-cadherin for survival of hES cells growing on LN-521 and clonal survival of human ES cells on LN-521/E-cadherin substratum. (a) Inhibition of hES cell adhesion by E-cadherin function blocking antibodies 1 h after plating on LN-521 at a density of 30,000 cells per cm−2. Bars represent adhesion of control HS181 hES cells treated with mouse IgG (IgGM) taken as standard value to compare and adhesion of the cells treated with 1 μg ml−1of the antibody (aE-cad). Error bars show s.e.m. (n=4). (b) Inhibition of hES cell survival on LN-521 coating by E-cadherin function blocking antibodies 24 h after plating at a density of 30,000 cells per cm2. Scale bars represent survival of control HS181 hES cells treated with mouse IgG (IgGM) taken as standard value to compare and survival of the cells treated with 1 μg ml−1of the antibody (aE-cad). Error bars show s.e.m. (n=4).Pvalue was calculated by Student’st-test: ***P<0.002. (c) Clonal density cultures of human ES cells 5 days after plating on LN-521/E-cadherin mixture in mTeSR1 medium with additional albumin. Almost all colonies were positive for alkaline phosphatase (ALP). Magnification × 5. Scale bar, 250 μm. (d) Ratios of ALP+colonies to the number of plated cells on Matrigel (Mg), LN-511 (LN511), LN-521 (LN521), E-cadherin (E-cad), Vitronectin/E-cadherin, LN-511/E-cadherin and LN-521/E-cadherin mixtures taken at 9:1 w/w ratio at a density of 150 cells per cm2. The cells were plated in mTeSR1 and mTeSR1 supplemented with additional albumin (letter A in parenthesis). Control cells were treated with Y-27632 (ROCK inhibitor, R) and plated in mTeSR1 with additional albumin (Mg(R, A)). Error bars show s.e.m (n=4).Pvalue was calculated by Student’st-test: ***P<0.002. (e) Cloning of HS980 and HS1001 cells plated at a density of 150 cells per cm2. Error bars show s.e.m (n=4). Figure 4: Importance of E-cadherin for survival of hES cells growing on LN-521 and clonal survival of human ES cells on LN-521/E-cadherin substratum. ( a ) Inhibition of hES cell adhesion by E-cadherin function blocking antibodies 1 h after plating on LN-521 at a density of 30,000 cells per cm −2 . Bars represent adhesion of control HS181 hES cells treated with mouse IgG (IgGM) taken as standard value to compare and adhesion of the cells treated with 1 μg ml −1 of the antibody (aE-cad). Error bars show s.e.m. ( n =4). ( b ) Inhibition of hES cell survival on LN-521 coating by E-cadherin function blocking antibodies 24 h after plating at a density of 30,000 cells per cm 2 . Scale bars represent survival of control HS181 hES cells treated with mouse IgG (IgGM) taken as standard value to compare and survival of the cells treated with 1 μg ml −1 of the antibody (aE-cad). Error bars show s.e.m. ( n =4). P value was calculated by Student’s t -test: *** P <0.002. ( c ) Clonal density cultures of human ES cells 5 days after plating on LN-521/E-cadherin mixture in mTeSR1 medium with additional albumin. Almost all colonies were positive for alkaline phosphatase (ALP). Magnification × 5. Scale bar, 250 μm. ( d ) Ratios of ALP + colonies to the number of plated cells on Matrigel (Mg), LN-511 (LN511), LN-521 (LN521), E-cadherin (E-cad), Vitronectin/E-cadherin, LN-511/E-cadherin and LN-521/E-cadherin mixtures taken at 9:1 w/w ratio at a density of 150 cells per cm 2 . The cells were plated in mTeSR1 and mTeSR1 supplemented with additional albumin (letter A in parenthesis). Control cells were treated with Y-27632 (ROCK inhibitor, R) and plated in mTeSR1 with additional albumin (Mg(R, A)). Error bars show s.e.m ( n =4). P value was calculated by Student’s t -test: *** P <0.002. ( e ) Cloning of HS980 and HS1001 cells plated at a density of 150 cells per cm 2 . Error bars show s.e.m ( n =4). Full size image Table 1 Cloning of individualized HS181 and HS980 cells on 96-well plates. Full size table LN-521/E-cadherin coating could also facilitate long-term self-renewal of hES cells. HS181 cells after 20 passages on the coating proved to be pluripotent (both in vitro and in vivo assays) and karyotypically normal ( Supplementary Fig. 8 ). The cells expressed stable and high levels of Oct4, Nanog, and Sox2, which was confirmed by immunostaining, fluorescence-activated cell sorting (FACS), and quantitative reverse transcriptase polymerase chain reaction ( Supplementary Fig. 8 ). Derivation of hES cell lines on LN-521/E-cadherin matrix Using LN-521/E-cadherin coating and TeSR2 medium supplemented with recombinant human serum albumin, we derived two new hES cell lines (summarized in Table 2 ) from ICMs. By now, HS916 and HS975 cells have been cultured for 20 and 40 passages, respectively ( Fig. 5a ). Pluripotency and karyotypic stability of HS916 was confirmed after 10 passages in xeno-free and defined conditions ( Fig. 5c–f ). Both lines expressed markers of pluripotency Oct4, Nanog, Sox2 and SSEA-4 as shown by immunostaining and FACS analysis ( Fig. 5a,b ). Moreover, three additional hES cells lines (HS980, HS999 and HS1001) were successfully derived from ICMs of six embryos on LN-521/E-cadherin matrix in chemically defined and xeno-free medium NutriStem hESC XF expressing markers of pluripotency Oct4, Nanog and Sox2 ( Fig. 5a ). The new cell lines were further characterized as described in Supplementary Table 1 . Table 2 Summary of new hES cell line derivation experiments. 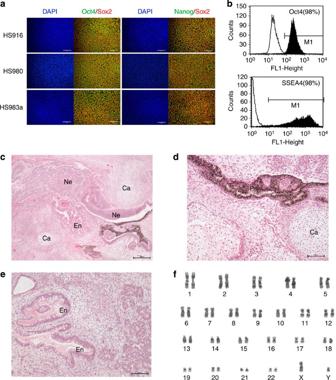Figure 5: Characterization of new human ES cell lines. (a) Immunostaining of the cells with anti-Oct4 (depicted as Oct4), anti-Nanog (Nanog), anti-Sox2 (Sox2) antibodies and DAPI. Scale bars, 100 μm. (b) FACS analysis of HS916 cells after 10 single-cell suspension passages on LN-521 in TeSR2 medium for Oct4 and SSEA4 (markers of pluripotency). The percentage of positive cells is listed in parentheses. (c–e) Pluripotency of teratoma forming HS916 hES cells after 10 passages (2 months) in culture. HE stained paraffin section of a teratoma shows features of various differentiating tissue lineages: Ne-neuroectodermal, with P representing pigmented neuroectodermal resembling retinal pigment epithelium; En-endodermal, represented by tubules lined by a single epithelial layer including vacuolated cells resembling goblet cells and a finely flocculent intratubular product consistent with mucin; Ca-cartilage, indicating mesodermal differentiation. Scale bars: in (c) 250 μm, in (d,e) 100 μm. (f) Karyotyping of HS916 cells after 10 single-cell suspension passages onto LN-521 in xeno-free chemically defined conditions. No chromosomal abnormalities were observed. Full size table Figure 5: Characterization of new human ES cell lines. ( a ) Immunostaining of the cells with anti-Oct4 (depicted as Oct4), anti-Nanog (Nanog), anti-Sox2 (Sox2) antibodies and DAPI. Scale bars, 100 μm. ( b ) FACS analysis of HS916 cells after 10 single-cell suspension passages on LN-521 in TeSR2 medium for Oct4 and SSEA4 (markers of pluripotency). The percentage of positive cells is listed in parentheses. ( c – e ) Pluripotency of teratoma forming HS916 hES cells after 10 passages (2 months) in culture. HE stained paraffin section of a teratoma shows features of various differentiating tissue lineages: Ne-neuroectodermal, with P representing pigmented neuroectodermal resembling retinal pigment epithelium; En-endodermal, represented by tubules lined by a single epithelial layer including vacuolated cells resembling goblet cells and a finely flocculent intratubular product consistent with mucin; Ca-cartilage, indicating mesodermal differentiation. Scale bars: in ( c ) 250 μm, in ( d , e ) 100 μm. ( f ) Karyotyping of HS916 cells after 10 single-cell suspension passages onto LN-521 in xeno-free chemically defined conditions. No chromosomal abnormalities were observed. Full size image Since our LN-521/E-cadherin matrix allowed clonal expansion and survival of hES cells, we explored if it could replace feeders and undefined components for clonal hES cell line derivation. Three different derivation protocols were tested of which one worked ( Table 3 ). Surplus frozen human cleavage stage embryos were thawn and incubated in G1 Plus cleavage medium for 24 h to the 8–10 cell stage under standard culture procedures. Multiple blastomere biopsies were obtained from each embryo to minimize the number of embryos used. For the successful protocol, six blastomeres were initially plated on a LN-521/E-cadherin matrix under oil in a 20 μl drop of G1 Plus medium supplemented with LN-511, LN521 and 20 mg ml −1 human recombinant serum albumin. The following day, four out of six blastomeres had attached, all of them having divided at least once. Subsequent feeding was done according to the protocol described in Table 3 Protocol N2. Four days after plating, three blastomeres gave small tight outgrowths of cells. Two weeks after the initial plating, one of them looked like a colony of human pluripotent cells, while two others had not survived. The former gave a stable HS983a line that expressed the pluripotency markers Oct4, Nanog and Sox2 ( Fig. 5a ). Since in our hands hES cells grew better in the xeno-free chemically defined NutriStem hESC XF medium, starting from the third week the TeSR2 medium was gradually changed to NutriStem XF. By now, HS983a has been passaged 20 times (4 months in culture). Its pluripotency was confirmed by in vitro assay ( Supplementary Fig. 7b ). Other groups of blastomeres that were fed according to the protocols described Table 3 , Protocols N1 and N 3 yielded no new hES cell lines. Previously, Klimanskaya et al. [21] and others [22] , [38] have reported derivation of new human ES cell lines from single blastomeres on feeder layers or undefined matrix in environments containing products of animal origin. Table 3 Experimental procedures for single blastomere derivation into new hES cell lines. Full size table Genetic analysis of DNA of newly derived hES cell lines To assess the genetic stability of newly derived lines, we performed karyotypic analyses of hES cell lines HS983a, HS975, HS980, HS999 and HS1001 ( Table 2 ) cells after 15, 35, 36, 10 and 12 passages, respectively. HS983a, HS980, HS999 and HS1001, similar to HS916 p.10 ( Fig. 5f ), had normal karyotypes ( Supplementary Fig. 9a–d ). Although, later in one of the cell culture branches HS983a cells acquired an abnormal male karyotype with an isochromosome 20q ( Supplementary Fig. 9e ). Out of 12 metaphases analysed of the HS975 line, 10 had a normal female karyotype and 2 had trisomy of chromosome 8 ( Supplementary Fig. 9f,g ). We carried on by performing genotyping of our cells at different time points of the experiment. Copy number variations (CNVs) and copy number neutral loss-of-heterozygosity (LOH) regions were analysed using Affymetrix Genome-Wide Human SNP Array 6.0 arrays and Genotyping Console Software version 4.1 (Affymetrix, Santa Clara, CA). The analysis was done by comparing each sample against a reference set of 75 healthy individuals (39 males, 36 females; genomic DNA extracted from blood ( n =61) or saliva ( n =14)). The minimum size of CNV segments was 50 kb. All samples fulfilled the general QC criteria recommended by Affymetrix ( Supplementary Table 2 ). In HS999 p.10, HS1001 p.15, HS980 p.31 and HS916 p.17, we detected 0, 3, 2 and 5 CNVs, respectively ( Supplementary Fig. 10a–c ). In HS983a p.15 cells, we did not detect any major abnormalities with only 1 CNV ( Supplementary Fig. 10c ). In control hES cells cultured on feeders HS401 p.25 and H1 p.56, we detected 1 and 3 CNVs ( Supplementary Fig. 10d ). Moreover, 1–4 CNVs could be detected even in some control samples from healthy individuals ( Supplementary Fig. 10e–h ). The ‘Y-chromosomal’ CNV segment in Yp11.2 seen in female samples HS999, HS980 and HS975 reflected X-Y homology rather than a stem-cell-related abnormality, since a similar segment was observed in all female reference samples (four shown in Supplementary Fig. 10e,f ). Some of newly derived male lines (HS1001, HS916 and HS983a) along with 12 out of 39 male reference samples had a CNV in Xq21.31 suggesting that it is either a common structural variant in a human population or it reflects X-Y homology in males rather than an abnormality ( Supplementary Fig. 10g,h ). These two CNVs were excluded from the analysis. All the other CNVs found in newly derived lines and in the male reference samples are listed in Supplementary Data 1 . Abnormalities found in HS975 p.35 ( Supplementary Fig. 10b ) corresponded to those seen by conventional karyotyping ( Supplementary Fig. 9e,f ). The general number of LOH regions did not differ radically between the newly derived and control lines ( Supplementary Table 3 ). To determine if the detected abnormalities had been acquired during culture, we compared early and late passages of cells with detected CNVs (HS980, HS1001, HS975 and HS983a lines in Supplementary Fig. 10i–l ). The trisomy of chromosome 8 was probably a result of adaptation, but apart from that, the overall number of CNVs and LOHs ( Supplementary Table 3 ) did not differ. For our initial experiments, we used late passages of HS181 cells initially cultured on feeders and iPSC line CVTB1.2. To test if culturing on LN-521 and LN-521/E-Cadherin substrata introduced mutations, we compared number of CNVs and LOHs at the beginning of the experiment for cells from feeders and after extensive passaging on the new substrata ( Supplementary Fig.10m–o and Supplementary Table 3 ). The overall number of aberrations was similar in both cases, suggesting that the substrata did not induce high rate of mutations. The present study provides a robust method for the derivation and self-renewal of hES cell lines. This method can facilitate the development of cells lines for human cell therapy purposes. First, we produced human LN-521, that is located in stem cell niches, as a full size trimeric protein in HEK-293 cells. Second, it was demonstrated that a combination of LN-521 and E-cadherin when used as a sole cell culture matrix enables clonal proliferation at as high a rate as 10–20%, self-renewal and derivation of new hES cell lines under completely chemically defined, xeno-free conditions, without the addition of any inhibitors of anoikis. Both proteins are biologically relevant for pluripotent hES cells, as they are normally expressed by cells in the blastocyst ICM [26] , [39] and by cultured pluripotent hES cells [4] , [34] . This xeno-free procedure may be appropriate for the derivation of hES cells for use in regenerative medicine. Third, it was demonstrated that use of the LN-521/E-cadherin matrix enables expansion of a single cell isolated from an 8-cell IVF embryo without a need to destroy it. We have previously shown that human recombinant LN-511, which is expressed in the blastocyst inner cell mass, alone can support monolayer cultures and self-renewal of both mouse ES [7] and human pluripotent ES and iPS cells [4] . The present results show that LN-521 provides a more robust substratum for renewal of hES cells and additionally in combination with E-cadherin permits their efficient clonal expansion not enabled by LN-511. The reason for this remains unclear. The trimeric LN-511 and LN-521 isoforms only differ with respect to the nature of the β chain. The exact biological roles of the β1 and β2 chain containing isoforms in LN-511 and LN-521, respectively, are not known, but they are developmentally regulated [8] . Thus, LN-511 is present in the embryonic glomerular basement membrane, but it is substituted by LN-521 after birth. Inactivation of the laminin β2 chain gene ( LAMB2 ) causes abnormal function of the glomerular filtration barrier and nephrotic syndrome [40] as well as disturbs the development of functional neuromuscular junctions [41] . Although human ES and iPS cells can grow indefinitely in culture, they commonly undergo adaptive changes during prolonged passaging in vitro . This has been attributed to the nature of pluripotent stem cells themselves rather than culture conditions [42] . Apart from random mutagenesis, the changes commonly involve nonrandom gains of chromosomes 12, 17, 20 and X, or large fragments of these chromosomes. A recent comprehensive study of more than 120 lines of human pluripotent cells has revealed one important example of small non-random culture adaptation in 20q11.21, which encompasses locus BCL2L1 , an anti-apoptotic factor [42] . The changes show similarity to those found in tumours [43] and such cells should not be used in medical applications. This underlines a need for systematic genetic analysis of cultured human pluripotent cells with high resolution methods such as genotyping. We observed several examples of these adaptations in human ES cells derived elsewhere ( Supplementary Fig. 10d,m ) and in one of the cell culture branches of HS983a cells after passage 20 ( Supplementary Fig. 9e ). Human ES cell lines derived on a LN-521/E-cadherin matrix in this study that were analysed at passages 10 to 15 showed 0 to 4 random small CNVs ( Supplementary Data 1 ) but no large abnormalities. Similar number of CNVs of similar sizes could also be seen in control samples from healthy individuals ( Supplementary Data 1 and Supplementary Fig. 10e–h ). With regard to genetic stability, rapid multiplication of cultured pluripotent cells in the LN-521 system is an advantage. Indeed, thawing of a standard aliqout of frozen human ES cells usually gives ~100 thousand living cells. Ten passages in the LN-521 culture system yield 429 × 10 12 cells (see growth curve in Fig. 1c ). Assuming that one cell weighs 1 × 10 −12 kg, this equals 429 kg. Therefore, cultures beyond passage 10–15 are not practically needed in the LN-521 culture system. Since feeder cells express large amounts of growth factors, cytokines and even ECM proteins by themselves, their use for new hES cell line derivation might mask important molecular cues which are needed for ICM cells to become an established line of pluripotent cells. We have demonstrated here that standard growth factor cocktails that are used for the self-renewal of established hES cell lines, and the simple LN-521/E-cadherin matrix developed here are sufficient for the derivation, which is important from a scientific standpoint. Cloning of hES cells may greatly facilitate manipulations with their genomes and applications based on the use of FACS. Also, derivation of new hES cell lines from single blastomeres acquired through a single-cell biopsy from an 8-cell IVF embryo is intriguing as it enables development of cells without a need to destroy the parental embryo. Such a single-cell biopsy method is a standard routine in IVF clinics for preimplantation diagnostics in families with certain genetic diseases. The method described here may facilitate the generation of hES cell lines with different HLA types for stem cell banking. Human ES and iPS cell cultures All the earlier established hES cell lines and human iPS ChiPSW cell line were provided by Prof Hovatta. CVTB1.2 cell line was provided by Dr Hansson. hES cells and iPS cells were maintained in O3, mTeSR1 (STEMCELL Technologies), TeSR2 (STEMCELL Technologies), and NutriStem hESC XF (Biological Industries, Israel) media. O3 medium is a variant of mTeSR1, prepared essentially as we have described earlier [4] , but with pH adjusted to 7.35. For clonal culture of hES cells and for derivation of new hES cell lines in TeSR2 and NutriStem hESC XF, the medium was supplemented with 20 mg ml −1 of additional bovine (Sigma) or human recombinant serum albumin (3H Biomedical, Sweden). Prior that, the protein had been dialyzed three times against 10 volumes of DMEM-F12 medium 1.5 h each time, using 10-kDa dialysis units. Initially, cells of previously derived lines were transferred onto a LN-521 coating from a human feeder cell layer by careful scratching using a sterile knife with subsequent trypsinization, or the cells were trypsinized into single-cell suspension from a LN-511 coating. The cells were provided once a day with fresh medium prewarmed in an incubator for 1 h, except for the first day after plating. If 1:20–1:30 passaging ratios were used, cells were routinely passed once in 10–12 days by exposure to Trypsin/EDTA (GIBCO Invitrogen Corporation, Paisley, Scotland) for 5 min at 37 °C, 5% CO 2 . They were then gently pipetted to break into single-cell suspension and a Defined Trypsin Inhibitor (GIBCO Invitrogen) was added. The cell suspension was centrifuged at 25 rcf for 4 min, the supernatant was discarded, the cell pellet was resuspended in prewarmed O3 medium, and the cells were then passed through a 40 μm sieve. Subsequently, the cells were plated on new LN-521–coated dishes at a concentration of choice. Control cells of the same line were cultured on Matrigel (STEMCELL Technologies) and LN-511 as described previously [4] . To achieve the fastest multiplication of hES/iPS cell number, 1:10 passaging ratio was used. In this case, the cells were passaged every 5–6 days. For defined and xeno-free cultures, TeSR2 (STEMCELL Technologies) medium or NutriStem hESC XF with defined xeno-free TrypLESelect (GIBCO Invitrogen) enzyme were used. The cells were passed by exposure to TrypLESelect for 4–5 min at 37 °C, 5% CO 2 . Then, the enzyme was carefully aspirated and prewarmed TeSR2 medium was added. After that, the cells were gently pipetted to break into single-cell suspension, centrifuged, the supernatant was discarded and the cell pellet was resuspended in prewarmed TeSR2. The cells were then passed through a 40 μm sieve and plated on a fresh LN-521-coated dish. Cells of the human-induced pluripotency cell (iPSC) line ChiPSW were derived from lentivirally transduced human foreskin fibroblasts with OCT-4/SOX2/NANOG/LIN28 reprogramming genes [44] , [45] , [46] . Prior to cell culture and passaging experiments, the cells were confirmed to express pluripotency markers. RT–PCR analyses confirmed that the cells lacked expression of the viral transgenes. Pluripotency of the ChiPSW cells was shown by in vitro and in vivo experiments. The CVTB1.2 cells were developed by Emil Hansson in Prof Chien’s laboratory (Harvard Stem Cell Institute) and kindly provided for this study. Prior to these experiments, the cells were shown to express pluripotency markers Oct4/Nanog/Sox2/TRA-1-60/TRA-1-81, to lack expression of the viral transgenes, and the pluripotency of the cells was confirmed both by in vivo and in vitro differentiation studies. Cell culture dish coating Laminins : Tissue cell culture plates from Sarstedt were coated overnight at 4 °C with sterile solutions of laminins, such as human recombinant LN-521, all at a concentration of 30 μg ml −1 (5 μg cm −2 ). Laminins were obtained from BioLamina AB and were produced as described below. Control plates were coated with Matrigel according to the STEMCELL Technologies’ instructions. Prior to use, dishes were prewarmed in an incubator for 1 h, washed once with phosphate-buffered saline (PBS) and after that prewarmed stem cell medium was added. The remaining laminin solution could be reused at least once more. All the adhesion, survival and inhibition of survival experiments were carried out using fresh coating materials. LN-521/E-cadherin coating : Recombinant human E-cadherin Fc Chimera (E-cadherin) was purchased from R&DSystems. LN-521 and E-cadherin were taken at 9 to 1 w/w ratio with DPBS containg Ca++ and Mg++ used to dilute the proteins. Tissue culture plates were coated at +37 °C for 2 h at a concentration of 13.5 μg ml −1 (2.25 μg cm −2 ) LN-521 and 1.5 μg ml −1 (0.25 μg cm −2 ) E-cadherin. After that the plates were washed twice with DPBS containing Ca++ and Mg++ and, then, prewarmed stem cell medium of choice was added. Laminin-521 and other coating materials To obtain a full-length human laminin β2 chain cDNA, a 5.6 kb fragment was PCR amplified from a human liver cDNA library (BD Biosciences) using primers 5′-GTGGTACCCACAGGCAGAGTTGAC-3′ and 5′-GCTCTAGAGCTCTTCAGTGCATAGGC-3′ thus introducing artificial XbaI and KpnI cutting sites on the ends of the fragment. To decrease the error rate during the PCR amplification Phusion, a high-fidelity PCR Kit (Finnzymes) was used. Subsequently, the fragment was digested with XbaI and KpnI and subcloned into a pSK vector (Stratagene) digested with the same restriction endonucleases (pSKHLAMB2 plasmid). To verify integrity of the sequence, several clones of pSKHLAMB2 plasmid were sequenced. Sequencing was performed on an ABI PRISM310 Genetic Analyzer (Perkin Elmer) using ABI PRISM BigDyeTerminator Cycle Sequencing kit (PE Applied Biosystems). Only complete matches with the NCBI database human laminin β2 sequence were selected for further cloning. For expression of the human laminin β2 chain, the pSKHLAMB2 plasmid was digested with XbaI and KpnI and subcloned into an XbaI-KpnI treated pcDNA 3.1(+) vector (Invitrogen). Constructs used for expression of full-size human laminin α5 (HLN5Full.pcDNA construct) and γ1 (HG1 construct) chains have been described previously [11] . Full-size trimeric human recombinant LN-521 (available from BioLamina, AB, Stockholm was then generated following triple transfection of human embryonic kidney cells (HEK293, ATCC CRL-1573)) essentially as described for production of LN-511 [11] . For protein production, the HEK293 cells were cultured for up to six days in Dulbecco’s modified Eagle’s medium (DMEM) supplemented with GlutaMax I. The LN-521 molecules were affinity-purified using anti-FLAG matrix (Sigma) as described earlier, and then characterized using 3–8% ( Supplementary Fig. 1a ) and 4–15% gradient SDS–PAGE under reducing and nonreducing conditions. The protein was visualized using Sypro Ruby (Bio-Rad) protein staining and immunostaining of the chains on polyvinylidene difluoride membranes. To further characterize the protein, Western blot analysis with antibodies against the laminin α5, β2 and γ1 chains was performed ( Supplementary Fig. 1b ). Human recombinant LN-111 and LN-121 were produced similarly to LN-521 and shown by western and SDS–PAGE to contain the correct chains of predicted molecular sizes. If not otherwise stated, the corresponding mouse LN-111 (Invitrogen) is indicated as LN-111. Reagents and antibodies InSolutionTM LY 294002 (a specific Akt inhibitor), InSolutionTM Wortmannin (a specific PI3K inhibitor) and InSolutionTM PD 98059 (a specific MEK1/Erk inhibitor) were purchased from Calbiochem. Antibodies to phospho-Akt (#4060), total-Akt (#9272), phospho-Erk (#9101) and total-Erk (#9102) were obtained from Cell Signaling Technology. PathScan Phospho-Akt1 sandwich ELISA kit (#7160), PathScan total Akt1 sandwich ELISA kit (#7170), PathScan Phospho-Akt2 sandwich ELISA kit (#7048) and PathScan total Akt2 sandwich ELISA kit (#7046) were also purchased from Cell Signaling Technology. Antibodies to Calnexin (#ab10286) were obtained from Abcam. Function blocking antibodies to various integrin subunits, mouse isotype antibodies and α-dystroglycan were purchased from Millipore. Since function blocking antibodies to αV (MAB1980) and α6 (MAB1378) were presented in a solution with sodium azide before the inhibition of survival experiment, all the antibodies to α integrin subunits were dialyzed thrice against O3 medium for 2 h each time. Antibodies to Lutheran receptor and α-fetoprotein, as well as rat isotype control antibodies were obtained from R&D Systems. Antibodies to Oct4, Nanog, SSEA-4, smooth muscle actin and MAP-2 were purchased from Millipore. Immunofluorescence For immunofluorescence studies, ES cells were cultured and fixed in 8-well slide chambers (BD Biosciences) or 96-well plate wells by 4% paraformaldehyde, permeabilized by 0.1% Triton X and blocked by 10% bovine fetal serum (GIBCO Invitrogen Corporation) in PBS containing 0.1% Tween-20 (Sigma-Aldrich, St. Louis, http://www.sigmaaldrich.com ) for 1 h. Incubation with primary antibody was performed for 1.5 h at room temperature. Incubation with secondary antibody and 4',6-diamidino-2-phenylindole (DAPI, Molecular Probes) was performed for 40 min. Between incubations, the specimens were washed with 0.1% Tween-20 in PBS buffer three to five times. Specimens were preserved in a fluorescence mounting medium (Dako, Glostrup, Denmark), and observed under a fluorescence microscope (Leica, Heerbrugg, Switzerland). Real-time PCR quantification of different mRNAs Total RNA was isolated using Absolutely RNA Microprep Kit (Stratagene, La Jolla CA, www.stratagene.com ) according to the manufacturer’s instructions. cDNA was synthesized using 0.2 μg of total RNA in 20 μl reaction mixture, containing oligo(dT)12–18 primers and Superscript II reverse transcriptase (GIBCO Invitrogen), according to the manufacturer’s instructions. Real-time quantitative RT–PCR Taqman assays were performed using the Applied Biosystems 7300 Real-Time PCR System (Applied Biosystems, Foster City, CA). All reactions were done in quadruplicates with the use of a pre-developed gene expression assay mix (Applied Biosystems) containing primers and a probe for the messenger RNA of interest. Additional reactions for each experiment included predeveloped gene expression assay mix for GAPDH for normalizing the RNA input. All data were analysed with 7300 System SDS Software v 1.4. FACS analysis Cells were removed from the culture dish with trypsin/EDTA, dissociated into single-cell suspension and resuspended in ice-cold FACS buffer (2% fetal bovine serum, 0.1% sodium azide in Hank’s buffer). Incubation with primary antibodies against SSEA-4 (from Millipore, Billerica) was performed for 1 h on ice. Then, the cells were washed three times with ice-cold FACS buffer. Subsequently, the cells were probed in FACS buffer with 1:400 dilution of Alexa Fluor anti-mouse secondary antibodies (GIBCO Invitrogen) for 30 min in the dark, and washed four times. Control cells were incubated with mouse immunoglobulins and, subsequently, with the secondary antibody as described above. Cells were analysed on FACSCalibur Flow Cytometer (Becton Dickinson, San Jose, CA). Data were analysed with the CellQuest software (Becton Dickinson). The analysis of Oct4 expression was performed as described previously [24] . Karyotyping Karyotyping of the cell lines was carried out using standard Q-banding techniques. Samples of cells were treated with colcemid KaryoMAX (0.1 mg ml −1 ; Gibco Invitrogen) for up to 5 h, followed by dissociation with trypsin/EDTA solution (Gibco Invitrogen). The cells were pelleted via centrifugation and resuspended in prewarmed 0.0375 M KCl hypotonic solution and incubated for 10 min. Following centrifugation, the cells were resuspended in fixative (3:1 methanol:acetic acid). Metaphase spreads were prepared on glass microscope slides and G-banded by brief exposure to trypsin and stained with 4:1 Gurr’s/Leishmann’s stain (Sigma-Aldrich). A minimum of 10 metaphase spreads were analysed and additional 20 were counted. In vivo imaging and migration assay Twenty-four well plates were coated with extracellular matrix proteins and blocked by O3 medium containing bovine serum albumin. The ES cells were plated at cell density of 30,000 cells per cm 2 onto extracellular matrix-coated plates and left to adhere for half an hour in a cell incubator. After that, the plates were transferred into a high throughput imaging system (Operetta PerkinElmer) equipped with an environmental control unit (37 °C, 5% CO 2 ). For Supplementary Movies 1 and 2 , the brightfield images were taken once in 15 min during 24 h after plating using Harmony software (PerkinElmer), exported and analysed using ImageJ software (NIH, the United States). For Supplementary Movie 3 , the images were taken once in 30 min for 5 days. For migration assays, the images were taken every 7 min. Images acquired between the fifth and seventh hours after plating were analysed using MTrackJ plug-in (University Medical Center, Rotterdam, The Netherlands). Hundred attached cells on each coating were traced and mean distances from the current to the previous point of the track were calculated. Error bars show standard error of the mean (s.e.m.) ( n =100). Teratoma formation Teratoma formation experiments were done as described before [47] , [48] by implantation of ~10 6 cells beneath the testicular capsule of a young (7-week-old) severe combined immunodeficiency SCID mouse or by injecting the cells subcutaneously in female SCID mice. Three–four animals were used for each cell line. Teratoma growth was observed by weekly palpation, and the mice were killed 8 weeks after the implantation. The teratomas were fixed, and sections were stained with hematoxylin and eosin or with hematoxylin, eosin and PAS. All animal experiments were performed at the infection-free animal facility of the Karolinska University Hospital in accordance with the ethical committee’s approval. Embryoid body formation ES cells from LN-521-coated cell culture dishes were exposed to DPBS (GIBCO Invitrogen) for 1 min at 37 °C, 5% CO 2 , washed two times with a medium, broken into large pieces and cultured in suspension in low adhesion plates. The medium used for this was Knockout DMEM (GIBCO Invitrogen) supplemented with 2 mM L -glutamine, 20% fetal calf serum (GIBCO Invitrogen), 0.1 mM β-mercaptoethanol (GIBCO Invitrogen) and 1% non-essential amino acids (GIBCO Invitrogen). After 1–2 weeks in suspension, the embryoid bodies were transferred onto gelatin-coated tissue cell culture 96-well plates (Sarstedt), cultured for 1–2 weeks, then fixed, stained with antibodies against markers of all three embryonic germ line layers (smooth muscle actin, MAP-2 and α -fetoprotein), and analysed as described above for immunofluorescence. Cell adhesion assay The assay was performed as described previously [7] . Briefly, 96-well plates were coated by extracellular matrix proteins as described above and blocked by O3 medium containing bovine serum albumin. The ES cells were plated at a density of 50,000 cells per cm 2 onto extracellular matrix-coated plates and left to adhere for 1 h in a cell incubator. Subsequently, the plates were washed three times with the medium to remove the non-adherent cells, and then the adherent cells were fixed for 20 min by 5% glutaraldehyde, stained by 0.1% Crystal Violet. (Kebo Lab, Spanga, Sweden). After 1 h and three washes with water, Crystal Violet was extracted with 10% acetic acid and quantified by measuring optical density at 570 nm. All the experiments were performed in quadruplicates. Cell survival and inhibition of survival assays The survival assay was performed as described for the cell adhesion assay above, except that the cells were left in the cell incubator for 24 h. For inhibition of the survival assay, the cells were kept in a medium with function blocking antibodies at the concentrations recommended by the manufacturer or pathway inhibitors at concentrations indicated in the text for 30 min, and then plated on the coated dishes. All the experiments were performed in quadruplicates. Western blotting and ELISA HS 181 cells were trypsinized into single-cell suspension as described above. For inhibition experiments, the cells were kept in O3 medium with blocking antibodies or pathway inhibitors for 30 min and then 450 K cells were plated on 35 mm dishes precoated with the appropriate matrix coating. For other experiments, same number of cells was plated directly after trypsinization. In all cases the cells were allowed to spread for 1 h at 37 °C, 5% CO 2 . After two washings in ice-cold PBS, plates with cells were snap frozen in liquid nitrogen and stored at −80 °C. To prepare samples for western blots and ELISA, the plates were slowly thawed and kept on ice with 100–150 μl of lysis buffer (50 mM Tris-HCl, pH7.5, 150 mM NaCl, 0.5% deoxycholate, 0.5% SDS, 1% Triton X-100, 1% Igepal, Complete (Roche) and Phospho-Stop (Roche)) on top. Then, the cells were scraped, pipetted and sheared through a 27G ¾′′ needle. After that, the cell pellets were clarified by centrifugation at 16,100 r.c.f. for 15 min at 4 °C. For western blots, 4–12% gradient gels were used for SDS electrophoresis and the proteins were transferred to polyvinylidene fluoride membranes. The membrane was hybridized with the antibody of interest according to the manufacturer’s instructions. Chemoluminescent HRP-substrate from Amersham Biosciences was used for visualization. For the densitometry analysis, the films were scanned at 2,400 d.p.i. and analysed by the ChemiImager5500 program (1D-Multi Line densitometry mode). For ELISA, the samples were applied to the wells according to the manufacturer’s instructions. Derivation of hES cell lines from whole ICMs of blastocysts The embryos for derivation of new ES cell lines were obtained as donations from the Fertility Unit of Karolinska University Hospital, Huddinge. Only embryos that could not be used for the couples’ infertility treatment were used after informed consent given by both partners of the couples. Both fresh and frozen–thawed supernumerary embryos were used. The work was done in accordance with ethics approval for derivation of new human ES cell lines issued to us by the Regional Ethics Board in Stockholm. Day 5–7 blastocysts donated after informed consent of both donors, were scored and transferred to 1.5 ml TESR2 (Stem Cell Technologies) or NutriStem hESC XF medium, in a 35 mm suspension culture plate (NUNC). Inner cell masses were isolated mechanically using two sharp metal needles (ICM tools were made of tungsten, provided by Hunter Scientific, Essex, UK). The blastocysts were held by one needle and dissected by the other under a stereo microscope (Nikon 1500). Then, the ICM was placed on LN521/E-cadherin matrix in a 20 μl drop of TESR2 (supplemented with 20 mg ml −1 of recombinant human albumin) or NutriStem hESC XF medium, under oil. After the derivation, the cells of new lines were passaged mechanically several times (to do that the cells were washed twice with DPBS, then DPBS was left on them for several minutes in an incubator, after that DPBS was replaced with prewarmed medium, the cells were carefully scraped using a pipette tip, and transferred to a new cell culture dish). After the adaptation period, the cells were passaged using the standard procedure of this study, that is, in single-cell suspensions with exposure to TrypLESelect (GIBCO) as described above. Derivation of new hES cell lines from single blastomeres The donated cleavage stage embryos, frozen 2 days after in vitro fertilization, were thawed using embryo thawing kit (Vitrolife, Gothenburg, Sweden) and cultured in G-1 Plus (Vitrolife) for 1 more day. Single blastomeres were biopsied in droplets of 30 μl biopsy medium G-PGD (Vitrolife) under mineral oil (Vitrolife). For a biopsy, the embryo was fixed by a holding pipette (Vitrolife) and the zona pellucida was pierced gently using a Saturn laser (The Saturn Active, Research Instruments, Cornwall, United Kingdom). One blastomere was acquired, immediately transferred to droplets containing fresh culture medium to be rinsed one time and, after that, placed on LN-521/E-cadherin matrix in a 20 μl drop of medium under oil. The work was done in accordance with ethics approval issued to us by the Regional Ethics Board in Stockholm. Three differentiation protocols were tested ( Table 2 ). Carrier free IL-6 and bFGF were purchased from R&D Systems and were reconstituted according to manufacturer’s instruction using triple dialyzed (as described above) human recombinant serum albumin. SNP 6.0 array CNVs and copy number neutral LOH regions were analysed using Affymetrix Genome-Wide Human SNP Array 6.0 array and Genotyping Console Software version 4.1 (Affymetrix, Santa Clara, CA). The analysis was done using default parameters and comparing each sample against a reference set of 75 healthy individuals (39 males, 36 females; genomic DNA extracted from blood ( n =61) or saliva ( n =14)) generated earlier in the same lab for a different project. The minimum size of CNV segments was five markers and 50 kb. Segments with 100% overlap with known CNV regions (according to the Toronto Database of Genomic Variants) were removed from the depicted results. All samples fulfilled the general QC criteria recommended by Affymetrix. Statistics Statistical significance was determined the by Student’s two-tailed t -test for unequal variances. Accession codes : SNP array data have been deposited in GEO database under accession number GSE53436 . How to cite this article : Rodin, S. et al. Clonal culturing of human embryonic stem cells on laminin-521/E-cadherin matrix in defined and xeno-free environment. Nat. Commun. 5:3195 doi: 10.1038/ncomms4195 (2014).